Evolutionary conservation of cold-induced antisense RNAs ofFLOWERING LOCUS CinArabidopsis thalianaperennial relatives Antisense RNA (asRNA) COOLAIR is expressed at A. thaliana FLOWERING LOCUS C ( FLC ) in response to winter temperatures. Its contribution to cold-induced silencing of FLC was proposed but its functional and evolutionary significance remain unclear. Here we identify a highly conserved block containing the COOLAIR first exon and core promoter at the 3′ end of several FLC orthologues. Furthermore, asRNAs related to COOLAIR are expressed at FLC loci in the perennials A. alpina and A. lyrata , although some splicing variants differ from A. thaliana . Study of the A. alpina orthologue, PERPETUAL FLOWERING 1 ( PEP1 ), demonstrates that AaCOOLAIR is induced each winter of the perennial life cycle. Introduction of PEP1 into A. thaliana reveals that AaCOOLAIR cis -elements confer cold-inducibility in this heterologous species while the difference between PEP1 and FLC mRNA patterns depends on both cis -elements and species-specific trans -acting factors. Thus, expression of COOLAIR is highly conserved, supporting its importance in FLC regulation. Many plant species growing in temperate climates flower in response to prolonged low winter temperatures, a process called vernalization [1] , [2] . In Arabidopsis thaliana FLOWERING LOCUS C ( FLC ) plays a central role in vernalization requirement, encoding a MADS box transcription factor that delays flowering until the plant is exposed to low temperatures [3] , [4] . On extended exposure to cold FLC mRNA level is progressively reduced, so that after several weeks it reaches trough levels [3] . On return to warmer temperatures, mimicking spring conditions, FLC repression is maintained and flowering occurs. Repression of FLC by cold involves epigenetic regulation. Histone modifications, particularly trimethylation of lysine 27 on histone 3 (H3K27me3), increase at FLC during vernalization through the activity of Polycomb Repressive Complex 2 (PRC2) and later spread across the gene [5] , [6] . This mechanism requires accessory components of the PRC2 that are cold-induced, such as PHD-finger protein VERNALIZATION INSENSITIVE 3 (VIN3) [7] , [8] , [9] . VIN3 as well as core PRC2 proteins such as VERNALIZATION 2 (VRN2) are required to maintain FLC in a repressed state after vernalization [7] , [9] , [10] . Repression of FLC is also proposed to involve long non-coding RNAs (lncRNAs) expressed at the locus in response to cold [11] . A sense lncRNA called COLDAIR is expressed during vernalization from a region in the long first intron [12] termed the vernalization response element (VRE) [13] . The VRE is downstream of the nucleation point at which chromatin modifications initially occur [5] and was previously shown to be important for stable silencing of FLC [13] , [14] . COLDAIR binds PRC2 components and promotes FLC stable repression [12] . Earlier during vernalization, before expression of COLDAIR, a set of alternatively spliced and polyadenylated antisense RNAs (asRNAs) termed COOLAIR are transiently expressed from the 3′ end of FLC [15] , [16] , [17] , [18] . Fusion of the COOLAIR promoter at the 3′ end of a green fluorescent protein (GFP) transgene can cause partial repression of GFP expression during vernalization [15] . COOLAIR has been shown to participate in FLC downregulation by the autonomous pathway but its function in the cold-induced silencing of FLC is still unclear [15] , [16] , [19] . Indeed, FLC marker genes lacking the COOLAIR promoter silence in cold [14] and FLC insertion alleles from which COOLAIR expression is not detectable are also silenced by vernalization [19] . Recently, COOLAIR transcription was shown to be downregulated by the formation of a RNA–DNA hybrid within its promoter. The so-called R-loop is stabilized by the homeodomain protein AtNDX (ref. 20 ). FLC homologues are found throughout the Brassicaceae family, of which A. thaliana is a member. Expression of some of these homologues has been shown to be reduced by vernalization [21] , [22] , [23] , [24] , [25] , [26] and genetic evidence demonstrates that some act as floral repressors [21] , [27] . In addition to their role in vernalization, differences in expression of FLC orthologues can contribute to diversification of life history within the Brassicaceae. A. thaliana is a representative monocarpic annual species of the family that flowers only once and then dies after seed set. However, other members of the family are polycarpic perennials and undergo multiple reproductive episodes during their life. Interestingly, in the perennial species Arabis alpina , A. halleri , Cardamine flexuosa and A. lyrata the expression patterns of FLC orthologues differ from A. thaliana FLC . The FLC genes in the perennials are not stably repressed by vernalization but their expression increases after return to warm temperatures [21] , [24] , [26] , [28] . The A. alpina FLC orthologue, PERPETUAL FLOWERING 1 ( PEP1 ), has additional perennial specific functions. For example, the increase in PEP1 mRNA after vernalization confers the return to vegetative growth after flowering until plants are exposed to low temperatures the following winter [21] . Comparison of transcriptional regulatory regions from several closely related species has been employed to identify conserved cis -regulatory elements in different taxa [29] , [30] , [31] including plants [32] , [33] , [34] . In contrast, the extent to which lncRNAs diverge during evolution has not been extensively analysed in plants, although in other systems such as mammals they appear to evolve rapidly between species [35] , [36] . To better understand what drives the conserved cold-regulation of FLC orthologues and to assess the functional significance of lncRNA at this locus, we combine phylogenetic shadowing of FLC cis -regulatory sequences with structural and temporal analysis of antisense transcription, especially at PEP1 , the best-characterized FLC orthologue. Our data reveal that the 3′ end sequences at FLC orthologues are more conserved than the 5′ promoter regions and that they promote antisense transcription at A. alpina PEP1 and A. lyrata FLC genes similar to what was observed in A. thaliana FLC . Introduction of PEP1 into A. thaliana shows that it contains all the cis -acting sequences required for cold repression and COOLAIR expression in this heterologous species. In contrast, the reactivation of PEP1 after vernalization seems to involve different trans -acting factors between A. alpina and A. thaliana. Evolutionary conservation of COOLAIR and its seasonal expression in perennial A. alpina supports a significant role for this asRNA in repression of FLC gene expression during vernalization. Conserved sequence blocks at the 3′ end of FLC orthologues In A. thaliana cold-induced repression of FLC mRNA requires cis -regulatory sequences in the promoter and first intron [13] , [14] . Whether these cis -regulatory elements are evolutionarily conserved was tested by comparing genomic sequences of FLC orthologues from a range of Brassicaceae species (Methods; Fig. 1 ; Supplementary Figs 1–3 ).With the exception of PEP1 in A. alpina , FLC orthologues from A. lyrata , Capsella rubella and Thellungiella halophila exhibit the same gene structure as A. thaliana FLC . A. alpina PEP1 harbours a tandem duplication ( PEP1a and PEP1b ) containing part of the promoter, the first exon and part of intron 1 ( Fig. 2a ; ref. 21 ). The two copies of exon 1 have individual transcriptional start sites and each is spliced to the unique exon 2 giving rise to two overlapping transcripts [37] . Two tandemly arranged full-length copies of FLC , called AlFLC1 and AlFLC2 , are present in A. lyrata , and both are transcriptionally active [26] , [38] . Promoter sequences between the translational start site (ATG) of FLC and the end of the next upstream gene were compared revealing two main blocks of homology ( Fig. 1a and Supplementary Fig. 1 ). The first block was ~400 bp long and included the proximal promoter as well as the 5′ untranslated leader. In A. alpina , homology in this region was reduced and mainly restricted to the untranslated leaders of PEP1a and PEP1b ( Supplementary Fig. 1g ). The second region was ~2 kb further upstream, and in A. alpina was found only in PEP1a . Apart from these two conserved blocks, the FLC promoter has diverged rapidly during evolution, even between the closely related species A. thaliana and A. lyrata , as observed previously [38] . 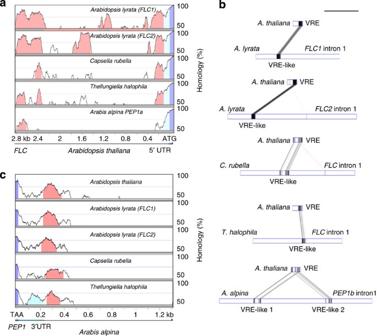Figure 1: Conservation and divergence of non-coding regulatorycis-elements amongFLCorthologues. (a) mVista pair-wise alignments of the 5′ intergenic regions ofFLCorthologues. From top to bottom,A. lyrata FLC1,A. lyrata FLC2,C. rubella FLC,T. halophila FLCandA. alpina PEP1aaligned toA. thaliana FLC. Alignment ofPEP1bandA. thaliana FLCis presented inSupplementary Fig. 1f. (b) GATA pair-wise alignment ofA. thalianaVRE to the first intron of each of theFLCorthologues mentioned ina. Regions showing homology to the VRE are annotated as VRE-like. ForA. alpina PEP1, VRE-like sequences were detected only in the region spanning exon 1b and exon 2 (intron 1 ofPEP1b). Scale bar, 1 kb. (c) mVista pair-wise alignment of the 3′ regions ofFLCorthologues.PEP13′ end was aligned to the 3′ intergenic regions ofA. thaliana FLC,A. lyrata FLC1,A. lyrata FLC2,C. rubellaandT. halophila FLCorthologues. Coloured areas in mVista graphs illustrate stretches of homology greater than 75% identity at the nucleotide level. Pink, regions of homology in the promoter region (a) or at the 3′ end (c); dark blue, exonic sequences; light blue, untranslated region. Grey and pink boxes in GATA plots are homologous regions and inverted homologous regions respectively (the darker the box, the higher the similarity). Figure 1: Conservation and divergence of non-coding regulatory cis -elements among FLC orthologues. ( a ) mVista pair-wise alignments of the 5′ intergenic regions of FLC orthologues. From top to bottom, A. lyrata FLC1 , A. lyrata FLC2 , C. rubella FLC , T. halophila FLC and A. alpina PEP1a aligned to A. thaliana FLC . Alignment of PEP1b and A. thaliana FLC is presented in Supplementary Fig. 1f . ( b ) GATA pair-wise alignment of A. thaliana VRE to the first intron of each of the FLC orthologues mentioned in a . Regions showing homology to the VRE are annotated as VRE-like. For A. alpina PEP1 , VRE-like sequences were detected only in the region spanning exon 1b and exon 2 (intron 1 of PEP1b ). Scale bar, 1 kb. ( c ) mVista pair-wise alignment of the 3′ regions of FLC orthologues. PEP1 3′ end was aligned to the 3′ intergenic regions of A. thaliana FLC , A. lyrata FLC1 , A. lyrata FLC2 , C. rubella and T. halophila FLC orthologues. Coloured areas in mVista graphs illustrate stretches of homology greater than 75% identity at the nucleotide level. Pink, regions of homology in the promoter region ( a ) or at the 3′ end ( c ); dark blue, exonic sequences; light blue, untranslated region. Grey and pink boxes in GATA plots are homologous regions and inverted homologous regions respectively (the darker the box, the higher the similarity). 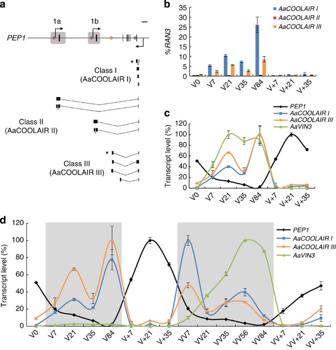Figure 2: Cold-induced antisense non-coding RNAs are transcribed at thePEP1locus inA. alpinaand follow a seasonal pattern. (a) Class I (AaCOOLAIR I), class II (AaCOOLAIR II) and class III (AaCOOLAIR III) antisense RNAs transcribed atPEP1locus. Black boxes are exons; lines are introns and other non-coding regions. Grey boxes indicate the region that is duplicated in tandem. Arrows indicate transcriptional start sites atPEP1. Dots showPEP1antisense transcript polyadenylation sites; blue, Class I; light orange, Class III; dark orange, Class II. Asterisks indicate the most abundant form among splicing variants obtained by 3′ RACE (Classes I and III) or RT–qPCR product sequencing (Class II). Scale bar, 1 kb. (b) AaCOOLAIR I, II and III cold-inducibility. RT–qPCR on leaf RNA ofA. alpinaplants exposed to 0, 7, 21, 35 and 84 days of vernalization (V0, V7, V21, V35 and V84) followed by 7, 21 and 35 days of growth in normal growth temperatures (V+7, V+21 and V+35). Transcript levels were expressed relative to those of the reference geneRAN3±s.d. (n=3 technical replicates). (c) AaCOOLAIR I, AaCOOLAIR III,PEP1andAaVIN3expression patterns inA. alpinaleaves during the vernalization time course shown inb. Transcripts levels were measured by RT–qPCR relative to those of the reference geneRAN3±s.d. (n=3 technical replicates). The maximum level of expression of each gene is set at 100%. (d) Seasonal expression patterns ofPEP1, AaCOOLAIR I, AaCOOLAIR III andAaVIN3over two successive vernalization treatments.A. alpinaplants were vernalized for 0, 7, 21, 35 and 84 days (V0, V7, V21, V35 and V84) followed by 7, 21 and 35 days of growth in normal temperature (V+7, V+21 and V+35), then vernalized again for 7, 21, 35, 56 and 84 days (VV7, VV21, VV35, VV56 and VV84) and grown for 7, 21 and 35 more days in normal growth temperatures (VV+7, VV+21 and VV+35). Grey areas indicate the cold treatments. Transcript levels were measured by RT–qPCR relative to those of the reference geneRAN3±s.d. (n=3 technical replicates). The maximum level of expression of each gene is set at 100%. A biological replicate is shown inSupplementary Fig. 8. Full size image Figure 2: Cold-induced antisense non-coding RNAs are transcribed at the PEP1 locus in A. alpina and follow a seasonal pattern. ( a ) Class I (AaCOOLAIR I), class II (AaCOOLAIR II) and class III (AaCOOLAIR III) antisense RNAs transcribed at PEP1 locus. Black boxes are exons; lines are introns and other non-coding regions. Grey boxes indicate the region that is duplicated in tandem. Arrows indicate transcriptional start sites at PEP1 . Dots show PEP1 antisense transcript polyadenylation sites; blue, Class I; light orange, Class III; dark orange, Class II. Asterisks indicate the most abundant form among splicing variants obtained by 3′ RACE (Classes I and III) or RT–qPCR product sequencing (Class II). Scale bar, 1 kb. ( b ) AaCOOLAIR I, II and III cold-inducibility. RT–qPCR on leaf RNA of A. alpina plants exposed to 0, 7, 21, 35 and 84 days of vernalization (V0, V7, V21, V35 and V84) followed by 7, 21 and 35 days of growth in normal growth temperatures (V+7, V+21 and V+35). Transcript levels were expressed relative to those of the reference gene RAN3 ±s.d. ( n =3 technical replicates). ( c ) AaCOOLAIR I, AaCOOLAIR III, PEP1 and AaVIN3 expression patterns in A. alpina leaves during the vernalization time course shown in b . Transcripts levels were measured by RT–qPCR relative to those of the reference gene RAN3 ±s.d. ( n =3 technical replicates). The maximum level of expression of each gene is set at 100%. ( d ) Seasonal expression patterns of PEP1 , AaCOOLAIR I, AaCOOLAIR III and AaVIN3 over two successive vernalization treatments. A. alpina plants were vernalized for 0, 7, 21, 35 and 84 days (V0, V7, V21, V35 and V84) followed by 7, 21 and 35 days of growth in normal temperature (V+7, V+21 and V+35), then vernalized again for 7, 21, 35, 56 and 84 days (VV7, VV21, VV35, VV56 and VV84) and grown for 7, 21 and 35 more days in normal growth temperatures (VV+7, VV+21 and VV+35). Grey areas indicate the cold treatments. Transcript levels were measured by RT–qPCR relative to those of the reference gene RAN3 ±s.d. ( n =3 technical replicates). The maximum level of expression of each gene is set at 100%. A biological replicate is shown in Supplementary Fig. 8 . Full size image Alignment of the intron 1 sequence of FLC with those of the orthologues showed that the extensive homology present in the closest species decreases in the more distantly related species until it is restricted to each end of the first intron and to the VRE ( Supplementary Fig. 2a–e ). These regions are important for FLC regulation by cold [13] , [14] . Sequences of the FLC orthologues showing homology to A . thaliana VRE were referred to as VRE-like and were found in all species examined ( Fig. 1b ). Interestingly, A . alpina PEP1 carries two VRE-like copies in intron 1, AaVRE-like 1 and AaVRE-like 2, both of which are located downstream of exon 1b. The COLDAIR promoter is contained within the most 5′ 100 bp of the VRE in A. thaliana [12] , [13] , and was the least conserved part of the VRE-like sequences, showing no detectable conservation even between A. thaliana and A. lyrata ( Fig. 1b and Supplementary Fig. 2a,b ). The FLC 3′ end harbours a promoter that drives the expression of the non-coding COOLAIR asRNA [15] . Alignment of the 3′ end of FLC to those of the orthologues showed strong conservation of a 150 bp block after the polyadenylation site ( Fig. 1c and Supplementary Fig. 3 ). Strikingly, this 3′ region is more widely conserved among the analysed species than either the 5′ intergenic region or first intron sequences implicated in FLC transcriptional regulation. In A. thaliana this evolutionarily conserved block is present within the COOLAIR first exon, the region bound by AtNDX to stabilize the R-loop and regulate COOLAIR expression [20] . Conservation of the 3′ ends of orthologous plant genes has not been extensively analysed, so to determine whether the conservation at this location of FLC is unusual, 10 other genes encoding MADS box transcription factors implicated in reproductive development were examined. The intergenic regions at the 3′ ends of orthologues from A. lyrata , C. rubella , T. halophila , A. alpina and A. thaliana were aligned ( Supplementary Fig. 4 ). For nine of the genes studied, conservation was observed only in the transcribed untranslated region present at the 3′ end of the cDNA, and this reduced steeply outside of the transcribed region, especially in more distantly related species. Therefore, strong conservation after the 3′ end of the transcribed region, similar to that present in FLC , is not detected among these genes. However, the remaining gene, SHATTERPROOF2 ( SHP2 ), exhibited conservation beyond the 3′ UTR that was similar to that observed for FLC . Interestingly, a potential natural antisense lncRNA is also annotated at its 3′ end and named At2g42835 ( Supplementary Fig. 4 ). Antisense transcription occurs at PEP1 3′ end The highly conserved 150-bp block present at the 3′ end of all FLC orthologues suggested that asRNAs might also be transcribed at these genes. The presence of antisense transcription was therefore tested at A. alpina PEP1 , the most characterized FLC orthologue. Several forms of PEP1 asRNA were detected by ‘3′ tiling’ RT–PCR and 3′ RACE PCR (see Methods and Fig. 2a ). The detected asRNAs were assigned to classes according to their structures and named based on the nomenclature used for A. thaliana COOLAIR [18] . Class I and II A. alpina PEP1 asRNAs have similar structures to those of A . thaliana COOLAIR [15] , [16] , [18] , and were named AaCOOLAIR I and AaCOOLAIR II, respectively. Class I asRNAs are polyadenylated within intron 6 of PEP1 , while those in Class II are spliced to a distal location in the PEP1 promoter. We further tested whether AaCOOLAIR II are polyadenylated within the promoter of PEP1a or PEP1b by making use of the accession Dorfertal (Dor), which contains polymorphisms in these regions [37] . Performing ‘3′ tiling’ RT-PCR for Dor PEP1 showed that class II asRNAs terminate in the promoter regions of both PEP1a and PEP1b ( Supplementary Fig. 5 ). A third class of PEP1 asRNA (AaCOOLAIR III) not documented in A. thaliana was also isolated, and is polyadenylated in intron 1 in a region that shows no homology with FLC ( Fig. 2a and Supplementary Fig. 2e ). We further confirmed the conservation of antisense transcription at the 3′ end of FLC orthologues by amplifying asRNA generated at A. lyrata FLC1 and FLC2 genes, both of which show homology to COOLAIR ( Fig. 1c ). Class I but not class II asRNA could be detected and harbour the typical splicing events of COOLAIR I asRNAs ( Supplementary Fig. 6a ). In contrast to the detection of asRNAs, non-coding sense RNA corresponding to COLDAIR could not be amplified at PEP1 after 5′ RACE PCR using several sets of primers downstream of the VRE-like 1 and the VRE-like 2 in intron 1 (5′ RACE ‘Tiling PCR’ in Supplementary Methods , Supplementary Table 1 ). Vernalized A. thaliana FRI SF FLC plants were also used as a control but the previously described COLDAIR transcript [12] could not be reliably detected, suggesting that our vernalization conditions or methodology may not be optimal for the detection of these non-polyadenylated transcripts. Therefore, COLDAIR could not be detected in A. alpina , but its presence cannot be excluded. Induction of AaCOOLAIR by cold in A. alpina The levels of the different AaCOOLAIR forms and their cold-inducibility were tested by RT–qPCR in A. alpina leaves during vernalization ( Fig. 2b ). AaCOOLAIR I and III were the most abundant forms. They showed two peaks of expression during cold exposure, after 21 and 84 days in the cold, and fell drastically when the plants were returned to higher temperatures after vernalization. Cold-inducibility seems to be reminiscent of class I asRNA at FLC orthologues as it was also observed for A. lyrata AlCOOLAIR I ( Supplementary Fig. 6b ). By contrast, class II asRNA could not be reliably amplified in A . lyrata . AaCOOLAIR II was detected but expressed at a very low level with no significant change in abundance during vernalization ( Fig. 2b ). In A. thaliana transcription of VIN3 is also induced during vernalization and is required for epigenetic silencing of FLC [7] . The A. alpina VIN3 orthologue was isolated based on sequence homology and showed conservation of synteny with A. thaliana ( Supplementary Fig. 7 ). AaVIN3 mRNA increased during cold, as observed in A. thaliana , and fell steeply at the end of vernalization ( Fig. 2c ). Seasonal cycling of AaVIN3 mRNA and AaCOOLAIR in A. alpina PEP1 expression repeatedly responds to seasonal changes in temperature contributing to the perennial life cycle of A. alpina [21] . Whether AaCOOLAIR I and III as well as AaVIN3 have similar responses was tested. A. alpina plants were exposed to two successive vernalization treatments separated by 35 days at normal growth temperatures. Leaves were harvested at regular time intervals during the treatment (see Methods). As expected, PEP1 mRNA levels responded to changes in temperature, being downregulated during cold and upregulated when plants were transferred to warm temperatures ( Fig. 2d , Supplementary Fig. 8 ). Interestingly, abundance of AaCOOLAIR I and III cycled inversely to PEP1 mRNA supporting the idea that they play a role in PEP1 repression. The timing of their maximal expression differed between the two cold treatments so that they reached peak level earlier in the second treatment than the first. AaVIN3 mRNA levels were dynamically induced by cold during both vernalization treatments presumably promoting PEP1 repression and the flowering of the plants during each following warm period ( Fig. 2c,d , Supplementary Fig. 8 ). Interestingly, the induction was more than 10-fold stronger during the second cold treatment than the first. Therefore, expression of AaCOOLAIR and AaVIN3 mRNA might be primed by the first vernalization treatment to respond more strongly during the second. PEP1b is stably silenced by cold in transgenic A. thaliana To investigate whether the molecular mechanisms regulating expression of FLC orthologues are evolutionarily conserved, A. alpina PEP1b ( Fig. 3a ), the most highly expressed A. alpina PEP1 gene [37] and the one containing the 3′ sequences encoding AaCOOLAIR, was transferred into A. thaliana Columbia FRI SF flc-3 (ref. 3 ). Transgenic FRI SF flc -3 plants containing the PEP1b genomic fragment displayed a small but statistically significant ( P <0.005) delay in flowering compared with the FRI SF flc -3 progenitor line ( Fig. 3b , Supplementary Table 2 ). By contrast, the control line FRI SF FLC that carries an active FLC gene flowered much later than FRI SF flc-3 ( Fig. 3b ). PEP1 mRNA was also expressed in FRI SF flc-3 PEP1b transgenic lines at lower levels than FLC mRNA in the FRI SF FLC control plants ( Fig. 3c , V0). These data suggest that the diverged PEP1b promoter might not be efficiently recognized in A. thaliana and cannot promote PEP1 mRNA at the threshold level necessary to strongly delay flowering time. To test the effect of cold on PEP1 mRNA level transgenic plants were vernalized for 40 days and subsequently transferred to warm temperatures for 20 days ( Fig. 3c ). PEP1 mRNA levels were reduced during vernalization as observed for FLC mRNA in FRI SF FLC control plants (V40, Fig. 3c ). Interestingly, in this heterologous species PEP1b mRNA level remained low when the transgenic plants were returned to normal growth temperatures after vernalization, similar to what is observed for FLC stable repression (V40+10, V40+20; Fig. 3c and Supplementary Fig. 9a ) and in contrast to the unstable repression of PEP1 found in A. alpina . However, the low level of expression of PEP1b in A. thaliana might also reduce the sensitivity of detection of reactivation after vernalization. Despite this reservation, the species-specific variation in trans -acting regulation is likely responsible for the differences in the stability of PEP1 repression observed between A. thaliana and A. alpina . 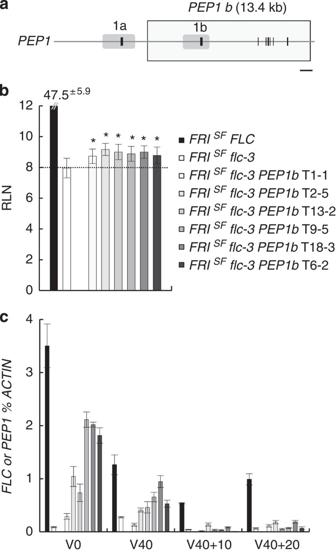Figure 3: Transcriptional activity ofPEP1binA. thaliana FRISFflc-3 PEP1btransgenic plants. (a) Schematic representation ofPEP1locus represented as described inFig. 2a. The rectangle indicates the extent of 13.4 kbPEP1btransgene transferred intoA. thaliana FRISFflc-3plants. Scale bar, 1 kb. (b) Flowering times ofA. thaliana FRISFflc-3 PEP1bindependent transformants,FRISFflc-3parental line andFRISFFLCcontrol line as measured by rosette leaf number (RLN) at bolting±s.d. (n=9–23 individuals). Asterisks indicate flowering time statistically different from the one ofFRISFflc-3plants (Student’st-test,Pvalue <0.005). (c)PEP1bmRNA levels inA. thaliana FRISFflc-3 PEP1bindependent transformants andFLCmRNA levels in the parentalFRISFflc-3line and the controlFRISFFLCline. Time points are before vernalization (V0), after 40 days of vernalization (V40), as well as after 40 days of vernalization followed by 10 or 20 days of growth at normal growth temperatures (V40+10 and V40+20). Transcript levels were measured by RT–qPCR relative to those of the reference geneACTIN±s.d. (n=3 technical replicates). Panelsbandcshare colour-code legends. Figure 3: Transcriptional activity of PEP1b in A. thaliana FRI SF flc-3 PEP1b transgenic plants. ( a ) Schematic representation of PEP1 locus represented as described in Fig. 2a . The rectangle indicates the extent of 13.4 kb PEP1b transgene transferred into A. thaliana FRI SF flc-3 plants. Scale bar, 1 kb. ( b ) Flowering times of A. thaliana FRI SF flc-3 PEP1b independent transformants, FRI SF flc-3 parental line and FRI SF FLC control line as measured by rosette leaf number (RLN) at bolting±s.d. ( n =9–23 individuals). Asterisks indicate flowering time statistically different from the one of FRI SF flc-3 plants (Student’s t -test, P value <0.005). ( c ) PEP1b mRNA levels in A. thaliana FRI SF flc-3 PEP1b independent transformants and FLC mRNA levels in the parental FRI SF flc-3 line and the control FRI SF FLC line. Time points are before vernalization (V0), after 40 days of vernalization (V40), as well as after 40 days of vernalization followed by 10 or 20 days of growth at normal growth temperatures (V40+10 and V40+20). Transcript levels were measured by RT–qPCR relative to those of the reference gene ACTIN ±s.d. ( n =3 technical replicates). Panels b and c share colour-code legends. Full size image Epigenetic regulation of PEP1 transgene in A. thaliana Whether A. alpina AaCOOLAIR was generated by mechanisms conserved in A. thaliana was examined. AaCOOLAIR was detected in the FRI SF flc-3 PEP1b transformants during vernalization ( Fig. 4a ), suggesting that trans -acting factors present in A. thaliana can promote AaCOOLAIR expression, including AaCOOLAIR III that is not found at FLC . In the control line FRI SF FLC , AtCOOLAIR I and AtCOOLAIR II were induced after 20 days in cold followed by accumulation of AtVIN3 mRNA and stable repression of FLC transcripts ( Fig. 4b ). Similarly, in transgenic FRI SF flc -3 PEP1b plants AaCOOLAIR I and AaCOOLAIR III were also induced by cold and their patterns of expression resembled those of A. thaliana COOLAIR I and II ( Fig. 4a,b ). Therefore, AaCOOLAIR transcripts are probably controlled by cis -regulatory elements present in PEP1 that are recognized by trans -acting factors conserved between A. thaliana and A. alpina. 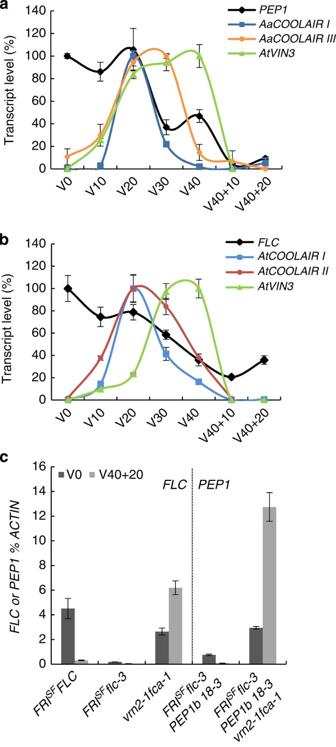Figure 4: Epigenetic control ofPEP1binArabidopsis FRISFflc-3 PEP1btransgenic plants. (a)PEP1b,AtVIN3and AaCOOLAIR I and III expression inFRISFflc-3 PEP1b 18-3transformant before vernalization (V0) after 10, 20, 30 or 40 days of vernalization (V10, V20, V30 or V40) and after 40 days of vernalization followed by 10 or 20 days of growth in normal temperature (V40+10, V40+20). (b)FLC,AtVIN3, AtCOOLAIR I and II expression inFRISFFLCcontrol plants during the vernalization time course described ina. InaandbmRNA levels were measured by RT–qPCR relative to those of the reference geneACTIN±s.d. (n=3 technical replicates) and presented relative to the maximum level of expression of each gene, which is set as 100%. (c)PEP1bmRNA level before vernalization (V0) and after 40 days vernalization followed by 20 days of growth at normal temperature (V40+20) inFRISFflc-3 PEP1b 18-3parental line andFRISFflc-3 PEP1b 18-3 vrn2-1 fca-1plants.PEP1bmRNA level is compared withFLCmRNA inFRISFFLC,FRISFflc-3andvrn2-1 fca-1plants. mRNA levels were measured by RT–qPCR relative to those of the reference geneACTIN±s.d. (n=3 technical replicates). Figure 4: Epigenetic control of PEP1b in Arabidopsis FRI SF flc-3 PEP1b transgenic plants. ( a ) PEP1b , AtVIN3 and AaCOOLAIR I and III expression in FRI SF flc-3 PEP1b 18 - 3 transformant before vernalization (V0) after 10, 20, 30 or 40 days of vernalization (V10, V20, V30 or V40) and after 40 days of vernalization followed by 10 or 20 days of growth in normal temperature (V40+10, V40+20). ( b ) FLC , AtVIN3 , AtCOOLAIR I and II expression in FRI SF FLC control plants during the vernalization time course described in a . In a and b mRNA levels were measured by RT–qPCR relative to those of the reference gene ACTIN ±s.d. ( n =3 technical replicates) and presented relative to the maximum level of expression of each gene, which is set as 100%. ( c ) PEP1b mRNA level before vernalization (V0) and after 40 days vernalization followed by 20 days of growth at normal temperature (V40+20) in FRI SF flc-3 PEP1b 18-3 parental line and FRI SF flc-3 PEP1b 18 - 3 vrn2-1 fca-1 plants. PEP1b mRNA level is compared with FLC mRNA in FRI SF FLC , FRI SF flc-3 and vrn2-1 fca-1 plants. mRNA levels were measured by RT–qPCR relative to those of the reference gene ACTIN ±s.d. ( n =3 technical replicates). Full size image In A. thaliana , FLC is stably silenced during cold by the deposition of chromatin-repressive marks (H3K27me3) and their spreading over the locus after return to normal growth temperature [6] , [39] , [40] , [41] . VRN2, a component of PRC2, is required for both establishing and maintaining this epigenetic silenced state [10] , [41] . To test whether chromatin modification by PRC2 is responsible for the stable repression of the PEP1b transgene observed in Arabidopsis FRI SF flc-3 PEP1b we investigated the effect of a vrn2 mutant allele on PEP1b expression. The vrn2-1 fca-1 mutations were introgressed into FRI SF flc-3 PEP1b background (see Methods). The fca-1 mutation impairs the autonomous flowering pathway and therefore increases FLC expression before vernalization but does not affect stable repression of FLC after vernalization [10] . FLC and PEP1 mRNA levels were measured in control and introgressed plants before and after 40 days of cold treatment ( Fig. 4c , Supplementary Fig. 9a ). The vrn2-1 fca-1 mutants failed to stably repress FLC mRNA expression upon vernalization, showing much higher FLC levels than in the FRI SF FLC control line 20 days after return to warm temperature ( Fig. 4c , V40+20). Such deregulation could also be observed for the residual endogenous FLC expression in FRI SF flc-3 PEP1b vrn2-1 fca-1 ( Supplementary Fig. 9b , V40+20). PEP1 mRNA levels in FRI SF flc-3 PEP1b vrn2-1 fca-1 transgenic lines were higher before vernalization compared with FRI SF flc-3 PEP1b 18-3 parental line ( Fig. 4c , V0), similar to what was described for the endogenous FLC in vrn2-1 fca-1 mutant [10] . Moreover, PEP1 showed a tremendous increase of expression 20 days after return to warm temperature in this background, whereas its mRNA levels were almost undetectable in FRI SF flc-3 PEP1b 18-3 parental line in which VRN2 is active ( Fig. 4c , V40+20). These data suggest that the stable repression of PEP1b observed in A. thaliana FRI SF flc-3 PEP1b transgenic lines is due to epigenetic silencing promoted by PRC2 either directly on PEP1b or indirectly by affecting expression of a trans-acting regulator. In this study, we demonstrate strong conservation of asRNAs expressed at FLC orthologues during vernalization in the related species A. alpina and A. lyrata . In perennial A. alpina we find that these asRNAs cycle in response to temperature changes through repeated vernalization treatments in a strictly inverse relationship to PEP1 mRNA, which argues for their involvement in the repression of FLC genes by cold. Phylogenetic shadowing combined with interspecies gene transfer showed that sequences required for transcriptional activation of FLC orthologues in A. thaliana and A. alpina have probably diverged, while variation in the stability of repression of these genes by vernalization is probably caused by trans -acting differences. These results provide insights into evolution of the structure and regulation of FLC , a gene that controls intra- and inter-species variation in flowering behaviour in Brassicaceae species. In A. thaliana and A. alpina , the orthologous genes FLC and PEP1 show different responses to cold. FLC is stably repressed by vernalization, whereas cold repression of PEP1 is unstable so that PEP1 mRNA levels increase again after return to warm conditions [21] . This difference in the stability of repression was not observed in transgenic A. thaliana carrying a genomic fragment of PEP1b , in which PEP1b mRNA stayed low after return to warm temperature. Introduction of a vrn2 mutation released PEP1b repression after return to warm conditions, suggesting that PEP1b stable repression is not caused by an inability to reactivate transcription. Thus, PEP1b must contain all the sequences required for an active process of stable repression in A. thaliana . The VRE and the COLDAIR lncRNA transcribed from it were previously shown to be required for stable silencing of FLC in A. thaliana [12] , [13] , [14] . We have shown that the VRE-like sequences present in PEP1b lack homology to the COLDAIR promoter. This divergence however does not impair PEP1b stable silencing in A. thaliana by a mechanism involving the PRC2 component VRN2. However, we cannot exclude that the effect of PRC2 on PEP1b in A. thaliana is indirect as H3K27me3 levels at the gene were not measured. The unstable PEP1 repression observed in A. alpina is most likely due to differences in the activity of trans -acting factors compared with A. thaliana and not to cis -acting differences such as those in the VRE, because PEP1b was stably repressed in A. thaliana , although the low level of expression of PEP1b in A. thaliana might also compromise our ability to detect reactivation. Trans -acting factors required for stable repression of FLC such as the components and accessory proteins of PRC2 (refs 7 , 8 , 10 , 41 ), LIKE HETEROCHROMATIN PROTEIN 1 (LHP1) or VERNALIZATION 1 (refs 13 , 42 , 43 ) are present in the A. alpina genome. Their absence, therefore, does not explain the instability of the H3K27me3 repressive marks at PEP1 (ref. 21 ). An alternative possibility is that A. alpina encodes enzymes that actively remove H3K27me3 from PEP1 allowing its reactivation after vernalization and that this activity is absent from annual A. thaliana . H3K27me3 demethylases are present in A. thaliana [44] , and members of this enzyme family might specifically target PEP1 after vernalization in A. alpina . PEP1b was only expressed at low levels in non-vernalized transgenic A. thaliana , suggesting that cis -regulatory elements required for PEP1b expression prior vernalization in A. alpina are not efficiently recognized in the heterologous species. Indeed, we found little 5′ homology between FLC and PEP1 , and what is present is restricted to a proximal block in PEP1a and PEP1b as well as a distal block only upstream of PEP1a . The latter is located 2 kb upstream of FLC translational start site in A. thaliana and outside the region shown to be sufficient for FLC regulation [14] . Other promoter regions moreover have been implicated in activation and repression of FLC expression [14] but did not exhibit high conservation in the PEP1 promoter. RNA or RNA polymerase-associated complexes have been described to be positive regulators of FLC expression [45] , [46] , [47] . These appear to act close to the transcriptional start site, which may explain the homology detected around this region. The proposed binding site of one of them, SUF4 (ref. 47 ), is however not conserved in PEP1. Also, one of two populations of A. lyrata studied by Kemi et al . [26] was monomorphic for a deletion in FLC1 promoter containing this binding site of SUF4. These findings further suggest that different mechanisms might promote PEP1 expression in A. alpina as well as FLC1 expression in A. lyrata. Our analysis demonstrated that the first introns of FLC orthologues, especially the flanks and the VRE-like sequences that are involved respectively in activating expression of FLC and stably repressing the gene in response to vernalization [12] , [13] , [14] , were generally more conserved than the promoter regions. In PEP1 these sequences might also contribute to its downregulation by cold although the VRE-like sequences present in the first intron do not confer stable repression in A. alpina . Both sense and antisense non-coding RNAs have been reported at FLC [12] , [18] . Similar to the FLC non-coding sense RNA COLDAIR, the HOTAIR non-coding sense RNA of humans was proposed to recruit PRC2 to the HOX gene cluster [48] , [49] . However, sequence comparisons and deletion of the mouse HOTAIR gene indicate that this regulatory function has diverged between humans and mouse [36] . Our phylogenetic shadowing approach showed that the COLDAIR promoter described in A. thaliana is not strongly conserved even in annual species in which FLC orthologues are stably repressed by cold. Additionally, we could not detect the sense COLDAIR RNA either in A. alpina or A. thaliana. These data raise the question whether this sense lncRNA is conserved in the Brassicaceae, but the absence of a reliable positive control prevents us from drawing a definitive conclusion. By contrast cold-inducible asRNAs were readily detected at FLC genes of A. lyrata and at PEP1 of A. alpina , respectively the closest and the most distantly related species to A. thaliana that we examined. The COOLAIR proximal promoter and the COOLAIR first exon at the 3′ end of all FLC orthologues were more highly conserved than most of the promoter region or first intron regulatory sequences of FLC . Such a high conservation was not observed at the 3′ ends of other MADS box genes, with the exception of SHP2 for which a potential natural antisense lncRNA is also annotated after the 3′ UTR. These analyses suggest that COOLAIR lncRNAs are under high constraint and likely have a role in cold repression of FLC . However, FLC derivatives lacking the 3′ end region or in which insertions prevent expression of COOLAIR still silence in the cold [14] , [19] , suggesting that COOLAIR is not essential for FLC silencing. Functional redundancy between COOLAIR and the VRE/COLDAIR might prevent detection of an effect of COOLAIR. Deletion of the VRE/COLDAIR prevents silencing but does not affect cold-mediated repression of FLC mRNA level [13] , so it would be interesting to test whether loss of both VRE/COLDAIR and COOLAIR prevents FLC downregulation in the cold. Nevertheless, current studies indicate that COOLAIR is not absolutely required for FLC cold-mediated repression or silencing, but might rather quantitatively enhance one or both of these processes. COOLAIR might also contribute more to FLC regulation in natural conditions where temperature and other environmental factors fluctuate widely. Mutations affecting flowering time were indeed previously shown to have different effects in natural conditions than in growth chamber experiments [50] . Studies of the A. thaliana fpa mutant, which is affected in polyadenylation signal recognition, suggest that the distal form of asRNA (COOLAIR II) might not play a role in FLC repression [16] , [17] . Our observation that the proximal COOLAIR I is the most conserved asRNA between A. thaliana , A. lyrata and A. alpina would support this hypothesis. The presence of distal asRNAs (AtCOOLAIR II, AaCOOLAIR II and III) may only be a consequence of inefficient polyadenylation at the termination site for Class I COOLAIR. Taken together our data suggest that Class I COOLAIR asRNAs are those with the major biological function and that their increased abundance during vernalization in A. thaliana , A. lyrata and A. alpina is a widely conserved feature associated with repression of FLC genes in cold. The polycarpic, perennial life cycle of A. alpina causes the plant to be exposed to vernalization many times during its life time, whereas annual, monocarpic A. thaliana is exposed to vernalization only once. We observed that PEP1 mRNA cycled with temperature, so that it was reactivated in the warm after vernalization [21] , and repressed again by a second vernalization treatment. AaCOOLAIR and AaVIN3 cycled in an inverse pattern to that of PEP1 . Interestingly, they appeared to be primed by the first vernalization treatment, resulting in a more rapid and enhanced rise in their expression during the second vernalization treatment. These differences suggest that perennial plants can maintain a memory of their first winter. Molecular mechanisms by which this occurs are unknown but might involve epigenetic changes or changes in chromosomal configuration. Such mechanisms are unlikely to involve increased H3K27me3 levels at PEP1 because this chromatin mark was shown to fall to pre-vernalization levels 3 and 5 weeks after cold treatment [21] . A gene loop occurring between FLC 5′ and 3′ regions is disrupted early during vernalization in A. thaliana . This chromosomal configuration change has been proposed to reveal COOLAIR promoter and favour its transcription [51] . Interestingly the pre-vernalized FLC 5′-3′ gene loop does not reform after return to warm temperature. Such a stable change in conformation might occur at PEP1 as well, and might provide a transcriptional memory responsible for COOLAIR priming. This could contribute to the increased sensitivity of older plants, which have already experienced a winter, to flower in response to inductive environmental conditions, a process often called competence to flower, which is particularly significant in perennials [52] . Analysis of sequences of FLC orthologues FLC sequences from A. lyrata , C. rubella and T. halophila (see Supplementary Data 1 for sequences) were obtained using genome browsers on phytozome ( www.phytozome.net ) and checking the synteny with A. thaliana . PEP1 genomic sequence was obtained from the BAC (accession number FJ543377.1). Pairwise alignments were performed using either Shuffle LAGAN [53] and visualized with VISTA browser using default settings [54] or with GATAliner (using default settings) and visualized with GATAplotter [55] . Plant material A. thaliana FRI SF FLC was obtained by introgression of the FRI allele of San-Feliu-2 into Columbia and FRI SF flc-3 was then recovered after EMS mutagenesis [3] . Transgenic lines FRI SF flc-3 PEP1b were obtained by floral dipping [56] of FRI SF flc-3 with the Agrobacterium carrying pGAP- PEP1b -Km plasmids (see Cloning) and confirmed by PCRs (primers set in Supplementary Table 3 ). FRI SF flc-3 PEP1b vrn2-1 fca-1 plants were obtained by crossing FRI SF flc-3 PEP1b 18-3 homozygote plants with vrn2-1 fca-1 double mutants [57] . A. alpina plants used in this study are from the Pajares and Dorfertal accessions [21] , [37] . Growth conditions Flowering time was measured on 9–23 plants per genotype ( Supplementary Table 2 ) grown in climate-controlled glasshouses (20 °C under long days, 16 h light per 8 h dark). A Student’s t -test was applied to determine whether the flowering behaviour of genotypes was statistically different from the control FRI SF flc3 with a P value <0.005. Vernalization experiments were carried out in A. thaliana plants grown 10 days in climate-controlled glasshouses (stratified 2 days at 4 °C), vernalized for 40 days at 4 °C under short days (8 h light per 16 h dark) and transferred back to climate-controlled glasshouses for 10 or 20 additional days. Full seedlings or rosette leaves were harvested before or after floral transition respectively. Fifty-six day old A. alpina plants grown in long days climate-controlled glasshouses (stratified 5 days s at 4 °C) were vernalized for up to 84 days at 4 °C under short days and transferred back to climate-controlled glasshouses for up to 35 additional days in long days. To mimic two successive winter periods, some of the A. alpina plants vernalized as described before were transferred for another 84 days at 4 °C under short days followed by 35 days in long days climate-controlled glasshouses. For each time point, one leaf of the same order was harvested from the main shoot on three different individuals. Cloning PEP1b cloning in the pGAP-Km vector was performed using the recombineering method [58] . The homology arms, EcoRI-Flank 1-SalI and SalI-Flank 2-BamHI were amplified by PCR (see Supplementary Table 3 for primers) on the PEP1 -BAC (FJ543377.1). After recombination in SW102 cells carrying PEP1 -BAC, the pGAP- PEP1b -Km was further extracted and transformed into Agrobacterium GV3101 (pPM90RK) strain. The introduced fragment was 13.4 kb comprising the 4.4 kb PEP1b 5′-intergenic region spanning the end of PEP1a upstream duplication to PEP1b , exon 1b to 7 and a 1.8 kb downstream segment harbouring the region of homology at the 3′ end of PEP1 and FLC . RNA extraction Total RNA was isolated using Trizol reagent (Invitrogen) and subsequently digested with DNAse I Amplification grade (Invitrogen) according to the manufacturer’s protocols. 3′ RACE PCR 3′ RACE experiments were performed on 3 μg of total RNA with the 3′ RACE System for Rapid amplification of cDNA ends (Invitrogen) according to the manufacturer’s protocol. PCR followed by a nested PCR were performed using AaCOOLAIR-specific forward primers (see Supplementary Table 3 ) together with the provided Universal Amplification Primer and the Abridge Universal Amplification Primer respectively. PCR products were cloned and sequenced. RT–qPCR and ‘3′ tiling’ RT–qPCR Reverse transcription was performed with oligo (dT) primers on 1 μg of total RNA using SuperScript II Reverse Transcriptase (Invitrogen) according to the manufacturer’s protocols. The qPCRs were performed on the Roche Light Cycler 480II instrument using the primer sets listed in Supplementary Table 3 and the IQ SYBR Green Supermix (Bio-Rad). Transcripts levels were expressed as a percentage of the accepted references genes RAN3 and ACTIN for A. alpina and A. thaliana samples respectively [12] , [21] . ‘3′ tiling’ RT–qPCR was used to approximately determine the 3′ end of AaCOOLAIR II transcripts. RTqPCRs utilizing the same forward primer but different reverse primers spanning the expected 3′ end of AaCOOLAIR II (see primer sets in Supplementary Table 3 ) were performed. Primers located progressively further towards the 3′ end were used until no amplification was detectable. PCR products were cloned and sequenced. How to cite this article: Castaings, L. et al . Evolutionary conservation of cold-induced antisense RNAs of FLOWERING LOCUS C in Arabidopsis thaliana perennial relatives. Nat. Commun. 5:4457 doi: 10.1038/ncomms5457 (2014).